Ih-mediated depolarization enhances the temporal precision of neuronal integration Feed-forward inhibition mediated by ionotropic GABA A receptors contributes to the temporal precision of neuronal signal integration. These receptors exert their inhibitory effect by shunting excitatory currents and by hyperpolarizing neurons. The relative roles of these mechanisms in neuronal computations are, however, incompletely understood. In this study, we show that by depolarizing the resting membrane potential relative to the reversal potential for GABA A receptors, the hyperpolarization-activated mixed cation current (I h ) maintains a voltage gradient for fast synaptic inhibition in hippocampal pyramidal cells. Pharmacological or genetic ablation of I h broadens the depolarizing phase of afferent synaptic waveforms by hyperpolarizing the resting membrane potential. This increases the integration time window for action potential generation. These results indicate that the hyperpolarizing component of GABA A receptor-mediated inhibition has an important role in maintaining the temporal fidelity of coincidence detection and suggest a previously unrecognized mechanism by which I h modulates information processing in the hippocampus. Microelectrode and electroencephalography studies show that groups of neurons can fire synchronously with millisecond precision [1] . To maintain temporal fidelity of information encoding, neurons act predominantly as coincidence detectors rather than neuronal integrators [2] . The precision of coincidence detection in pyramidal cells depends critically on feed-forward inhibition [3] , [4] . Such inhibition, mediated by GABA A receptors, acts both by shunting excitatory currents (shunting inhibition) and by hyperpolarizing neurons (voltage inhibition) [5] . Shunting inhibition reduces the amplitude and duration of excitatory postsynaptic potentials (EPSPs) by increasing the membrane conductance. The hyperpolarizing action of inhibitory postsynaptic potentials (IPSPs), on the other hand, offsets the depolarization mediated by EPSPs and is long lasting, resulting in a biphasic EPSP–IPSP sequence in many neurons [5] . It has been suggested that the temporal precision of neuronal integration also depends on I h , but this effect has been attributed to HCN-mediated shunting of excitatory inputs [6] . I h is a mixed cationic current with a reversal potential of ∼ −30 mV present in neurons throughout the brain (for reviews see refs 7 , 8 ). As I h is present at resting membrane potential, it depolarizes neurons [9] , [10] , [11] . I h has a marked effect on dendritic processing by directly shunting excitatory inputs [12] , [13] and through interactions with other membrane conductances [14] , [15] . Consequently, blocking I h facilitates the temporal summation of EPSPs and action potential firing during repetitive stimulation [12] , [13] , [16] . As I h can also affect IPSP kinetics [17] , [18] , we asked what effect I h blockade has on coincidence detection, when inhibition is left intact. Here, we report that blocking I h results in a significant broadening of the window for neuronal integration. This, however, is not due to the influence of I h on PSP kinetics, but rather is secondary to the hyperpolarizing effect of I h blockade. Indeed, I h is required to maintain the hyperpolarizing action of synaptically released GABA, and so, blocking I h broadens the excitatory phase of the EPSP–IPSP sequence evoked by afferent stimulation. These results show an essential role for I h in determining the relative values of the resting membrane potential ( V R ) and the reversal potential for GABA A receptor-mediated currents ( E GABA(A) ), and also show that hyperpolarizing inhibition is necessary for temporally precise neuronal integration of synaptic inputs. Blocking I h increases the integration time window We assessed coincidence detection by recording from CA1 pyramidal cells using gramicidin perforated-patch in current-clamp mode [19] . We stimulated two separate populations of Schaffer collaterals ( Fig. 1a ) representing weak and strong synaptic inputs (see Methods ). The stimulus intensities were adjusted so that simultaneous activation of the two pathways resulted approximately in a 50% chance of the neuron spiking. We then measured the spike probability while systematically varying the interstimulus interval. As previously reported, the spike probability decreased as the interval increased ( Fig. 1b,c ). We used 10 μM ZD-7288 to block I h . Again consistent with previous studies [9] , [10] , this resulted in a hyperpolarization, an increase in input resistance and complete disappearance of the characteristic depolarizing sag of the membrane potential following a hyperpolarizing step current injection ( Supplementary Fig. S1 ). We then readjusted the stimulation intensities to match the spiking probability for simultaneous stimulation observed under control conditions. Blocking I h resulted in a significant broadening of the time window for integration of the two input stimuli ( Fig. 1d–f ; n =6; repeated measures analysis of variance (ANOVA): F (1,5)=15.5, P =0.011). We further confirmed this effect using cell-attached recordings at near physiological temperature and with the same stimulation paradigm ( Supplementary Fig. S2 ; n =4; repeated measures ANOVA: F(1,3)=37.3, P =0.009 for the effect of ZD-7288). 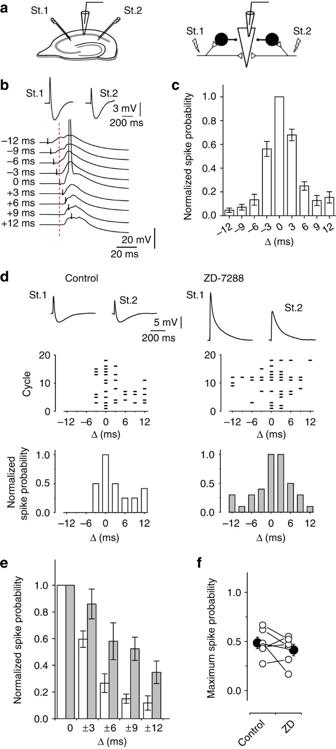Figure 1: Block of Ihwidens the coincidence-detection time window. (a) Two Schaffer collateral pathways (St.1 and St.2) were stimulated on either side of the recorded neuron∼300 μm away from the soma to evoke EPSP–IPSP sequences. (b) Both pathways were then activated at different interstimulus intervals. Traces show sample responses. Stimulation intensities were adjusted so that the probability of evoking action potential was 50% when the two stimuli were delivered simultaneously. (c) Summary graph of probability of evoking an action potential against the interval between stimulations (n=19). (d) Sample experiment demonstrating a change in the coincidence-detection time window following Ihblockade with ZD-7288. Top: Sample traces recorded in response to stimulation of two pathways in control and after application of ZD-7288; middle: raster plots of spike generation; bottom: frequency histograms showing spike probability at different intervals between stimuli. (e) Summary graph of relative probability of firing at different interstimulus intervals in control conditions (open columns) and in the presence of ZD-7288 (shaded columns;n=6;P=0.011 for difference). (f) The probability of evoking an action potential by simultaneous activation of both pathways under baseline conditions and after the readjustment of stimulus intensity following Ihblock (open circles: individual recordings; closed circles: averaged data;n=6). Error bars represent s.e.m. Figure 1: Block of I h widens the coincidence-detection time window. ( a ) Two Schaffer collateral pathways (St.1 and St.2) were stimulated on either side of the recorded neuron ∼ 300 μm away from the soma to evoke EPSP–IPSP sequences. ( b ) Both pathways were then activated at different interstimulus intervals. Traces show sample responses. Stimulation intensities were adjusted so that the probability of evoking action potential was 50% when the two stimuli were delivered simultaneously. ( c ) Summary graph of probability of evoking an action potential against the interval between stimulations ( n =19). ( d ) Sample experiment demonstrating a change in the coincidence-detection time window following I h blockade with ZD-7288. Top: Sample traces recorded in response to stimulation of two pathways in control and after application of ZD-7288; middle: raster plots of spike generation; bottom: frequency histograms showing spike probability at different intervals between stimuli. ( e ) Summary graph of relative probability of firing at different interstimulus intervals in control conditions (open columns) and in the presence of ZD-7288 (shaded columns; n =6; P =0.011 for difference). ( f ) The probability of evoking an action potential by simultaneous activation of both pathways under baseline conditions and after the readjustment of stimulus intensity following I h block (open circles: individual recordings; closed circles: averaged data; n =6). Error bars represent s.e.m. Full size image Blocking I h prolongs excitation through hyperpolarization Input summation in the above experiments depends on the time course of the EPSP–IPSP sequence [4] , [19] , [20] . The long membrane time constant of hippocampal principal cells permits EPSP summation over a large time window, but disynaptic feed-forward inhibition limits the temporal summation of the excitatory inputs by curtailing the EPSPs [4] , [19] . I h could influence the EPSP–IPSP sequence profile by altering membrane conductance [21] , [22] , interneuron recruitment [23] and/or V R [9] , [10] , [11] . To address the relative roles of these effects of I h , we evoked an EPSP–IPSP sequence in CA1 pyramidal cells by stimulating Schaffer collaterals, and then blocked I h with and without correcting the membrane voltage ( Fig. 2 ). Blocking I h with ZD-7288 completely abolished the hyperpolarizing component of the EPSP–IPSP sequence and resulted in considerable broadening of the half-width of the depolarizing phase of the response to 251±27% of control ( n =4; P =0.003; Fig. 2a,b ). 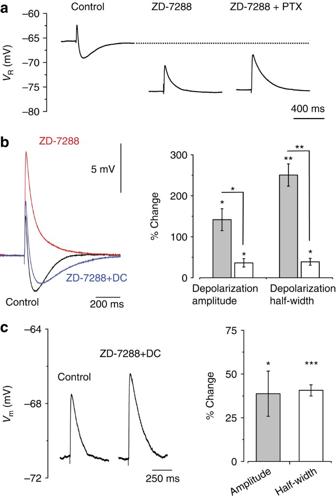Figure 2: Ihblock abolishes the hyperpolarizing phase of the EPSP–IPSP sequence. (a) EPSP–IPSP sequences were evoked in CA1 pyramidal cells by Schaffer collateral stimulation as inFigure 1. Consecutive traces from a representative experiment showing a shift inVRfollowing ZD-7228 application, associated abolition of the GABAAreceptor-mediated hyperpolarizing component of the EPSP–IPSP sequence (GABABreceptors are blocked with 5 μM CGP52432) and the overall contribution of inhibition revealed by subsequent application of picrotoxin (PTX). (b) Summary of ZD-7288 effect on EPSP–IPSP characteristics with (direct current (DC)) and without constant current injection to compensate for ZD-7288-induced shift inVR(n=4 cells; shaded columns: ZD-7288, open columns: ZD-7288+DC). Overlapped averaged traces are shown on the left (prepulse baseline is normalized). (c) Effect of application of ZD-7288 on the amplitude and duration of pharmacologically isolated EPSPs, while maintainingVRwith current injection (n=7; recordings were made in the presence of 5 μM CGP52432 and 100 μM picrotoxin); this effect is similar to the effect of ZD-7288 on the EPSP–IPSP sequence+DC (b). Bar charts represent percentage change of control values; error bars represent s.e.m.; *P<0.05, **P<0.01, ***P<0.001. Figure 2: I h block abolishes the hyperpolarizing phase of the EPSP–IPSP sequence. ( a ) EPSP–IPSP sequences were evoked in CA1 pyramidal cells by Schaffer collateral stimulation as in Figure 1 . Consecutive traces from a representative experiment showing a shift in V R following ZD-7228 application, associated abolition of the GABA A receptor-mediated hyperpolarizing component of the EPSP–IPSP sequence (GABA B receptors are blocked with 5 μM CGP52432) and the overall contribution of inhibition revealed by subsequent application of picrotoxin (PTX). ( b ) Summary of ZD-7288 effect on EPSP–IPSP characteristics with (direct current (DC)) and without constant current injection to compensate for ZD-7288-induced shift in V R ( n =4 cells; shaded columns: ZD-7288, open columns: ZD-7288+DC). Overlapped averaged traces are shown on the left (prepulse baseline is normalized). ( c ) Effect of application of ZD-7288 on the amplitude and duration of pharmacologically isolated EPSPs, while maintaining V R with current injection ( n =7; recordings were made in the presence of 5 μM CGP52432 and 100 μM picrotoxin); this effect is similar to the effect of ZD-7288 on the EPSP–IPSP sequence+DC ( b ). Bar charts represent percentage change of control values; error bars represent s.e.m. ; * P <0.05, ** P <0.01, *** P <0.001. Full size image We first examined whether the effect of I h block on the EPSP–IPSP sequence could be entirely accounted for by hyperpolarization of V R . Following the application of ZD-7288, V R was returned to the baseline level by injecting a constant current into the recorded neuron and the EPSP–IPSP sequence was again recorded ( Fig. 2b ). Almost full recovery of the hyperpolarizing phase of the response was observed (80±8% of the baseline amplitude before ZD-7288 application; n =4; P =0.1). In these experiments, there was only a relatively small increase in peak amplitude (36±10%; P =0.04) and half-width (39±9%; P =0.02) of the depolarization, consistent with some direct effect of I h on the EPSPs; these effects were significantly smaller than those observed with the addition of ZD-7288 without current injection (that is, without correcting the neuronal hyperpolarization; P =0.02 and P =0.004 for amplitude and half-width of depolarizing phase of the EPSP–IPSP sequence, respectively ( Fig. 2b )). The changes in the EPSP amplitude and half-width following ZD-7288 application and direct current injection ( Fig. 2b ) were similar to those observed when testing the effect of ZD-7288 on EPSPs when GABA A receptors were also blocked with 100 μM picrotoxin ( Fig. 2c , V R was fixed at the control level with direct current injections). These results argue against a significant contribution of non-specific effects of ZD-7288 on presynaptic function [24] . In addition, because of the limited space clamp in our experimental conditions (see Methods ), recovery of the hyperpolarizing component of the postsynaptic response by current injection indicates that the majority of the inhibitory synapses recruited by Schaffer collateral stimulation impinge either close to the soma or on proximal dendrites of pyramidal cells. This is in line with previous findings that feed-forward inhibition in hippocampal CA1 pyramidal neurons underlying temporally precise synaptic integration is predominantly perisomatic [4] . We further tested the effect of I h block on GABA A receptor-mediated transmission, as I h has been reported to be present in some interneurons [23] , [25] , [26] . We stimulated Schaffer collaterals and recorded in whole-cell voltage-clamp configuration with the membrane potential clamped to 0 mV (the reversal potential for glutamatergic currents) to isolate inhibitory postsynaptic current (IPSCs). Consistent with the results obtained in current clamp, ZD-7288 only reduced the IPSC amplitude by 17.5±3% ( n =3). The effect of I h on the EPSP–IPSP sequence can therefore be largely attributed to the I h -dependent depolarization of V R and to the loss of the hyperpolarizing action of the IPSPs. Does shunting inhibition also modify the EPSP–IPSP sequence? To test this, we applied the GABA A receptor antagonist picrotoxin with I h blocked. This resulted in further prolongation of the EPSPs, indicating an additional role of shunting inhibition in regulating the shape of the EPSP–IPSP sequence ( Fig. 2a ). One prediction from these results is that genetic ablation of I h should similarly hyperpolarize neurons, change the driving force for chloride and prolong the depolarizing phase of the EPSP–IPSP sequence. We examined HCN1 knockout mice and compared them with wild-type littermate controls. Consistent with previous studies [27] , [28] , HCN1 knockouts lacked the I h -mediated membrane potential sag following hyperpolarizing step current injection ( Fig. 3a ). The resting membrane potential of pyramidal cells was more hyperpolarized in the knockout mice (−72.6±2.5 mV) compared with wild-type littermate control animals (−61.9±1.6 mV; P =0.0037; Fig. 3a–c ); however, E GABA(A) was similar in both genotypes ( Fig. 3b,d ). As predicted, the hyperpolarizing phase of the EPSP–IPSP sequence was either absent or reduced in the knockout animals, and the width of the EPSPs was broadened to 193.4±18.4% of the wild-type value ( P =0.009; Fig. 3e ). 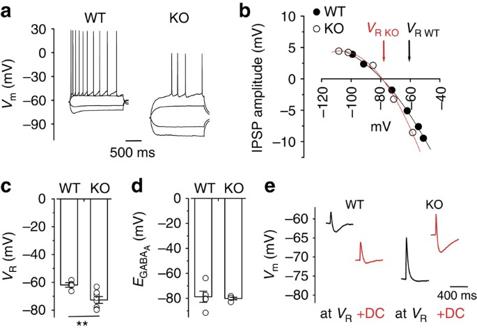Figure 3: HCN1 deletion results in the loss of the hyperpolarizing effects of GABAAreceptor-mediated inhibition. (a) Example traces showing voltage responses to current steps injections in wild-type (WT) mice and HCN1 knockout (KO) mice. (b) An example plot showing that, unlike WT mice, HCN1 KO mice lacked a hyperpolarizing GABAAreceptor-mediated driving force. Data points were fitted with a second-order polynomial function. (c) Comparison ofVRin HCN1 KO mice and WT mice (WT:n=5; KO:n=8). (d) Summary plot ofEGABA(A)in both genotypes (WT:n=5; KO:n=4). (e) Sample traces showing that the KO mice displayed no hyperpolarizing phase atVR, whereas WT animals had a biphasic EPSP–IPSP sequence. The hyperpolarizing IPSPs became apparent in the KO mice when cells were depolarized by DC injection. Conversely, the IPSP was less evident when pyramidal cells from WT mice were hyperpolarized. Error bars represent s.e.m.; **P<0.01. Figure 3: HCN1 deletion results in the loss of the hyperpolarizing effects of GABA A receptor-mediated inhibition. ( a ) Example traces showing voltage responses to current steps injections in wild-type (WT) mice and HCN1 knockout (KO) mice. ( b ) An example plot showing that, unlike WT mice, HCN1 KO mice lacked a hyperpolarizing GABA A receptor-mediated driving force. Data points were fitted with a second-order polynomial function. ( c ) Comparison of V R in HCN1 KO mice and WT mice (WT: n =5; KO: n =8). ( d ) Summary plot of E GABA(A) in both genotypes (WT: n =5; KO: n =4). ( e ) Sample traces showing that the KO mice displayed no hyperpolarizing phase at V R , whereas WT animals had a biphasic EPSP–IPSP sequence. The hyperpolarizing IPSPs became apparent in the KO mice when cells were depolarized by DC injection. Conversely, the IPSP was less evident when pyramidal cells from WT mice were hyperpolarized. Error bars represent s.e.m. ; ** P <0.01. Full size image I h maintains V R more depolarized than E GABA(A) The results thus far indicate that I h -dependent neuronal depolarization is necessary to maintain a hyperpolarizing effect of GABA A receptor currents. We directly tested this hypothesis using gramicidin perforated-patch current-clamp recordings, which minimize perturbation of the internal Cl − concentration. E GABA(A) was determined from the reversal potential of evoked IPSPs, and was uniformly negative to V R (mean E GABA(A) – V R : −5.2±1.0 mV; n =12; P =0.0003; Fig. 4a ). In all cells, application of ZD-7288 resulted in a significant negative shift in V R (−8.6±0.9 mV; P =7.4×10 −7 ; n =12; Fig. 4b,c ). In contrast, inhibition of I h led to only a small depolarizing shift in E GABA(A) (2.1±0.8 mV; P =0.03; Fig. 4d ). The net effect of blocking I h was to make V R more negative than E GABA(A) in 10 out of 12 cells (mean E GABA(A) – V R : 5.5±1.3 mV; n =12; P =0.0013; Fig. 4e ). This demonstrates a major role of I h in maintaining a hyperpolarizing driving force for fast GABAergic transmission. 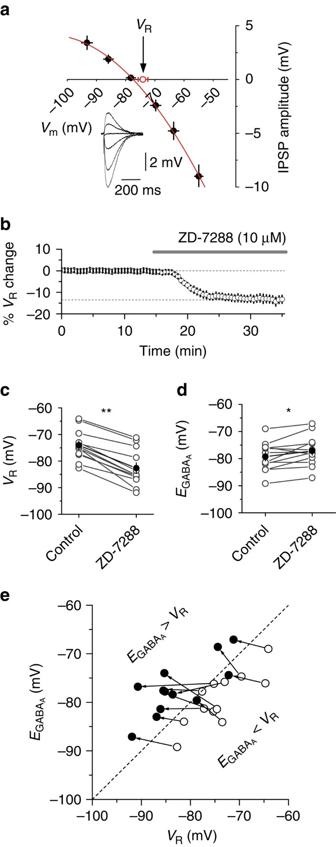Figure 4: Blocking Ihchanges theVR–EGABA(A)relationship in CA1 pyramidal cells. (a) In control conditions, all cells had negativeEGABA(A)compared withVR(n=12). Sample IPSPs at different membrane potentials from a typical experiment are shown in the inset. Data points were fitted with a second-order polynomial function. (b) Time course of the changes inVRfollowing the application of ZD-7288 (n=12). (c) Effect of ZD-7288 onVR(filled circles are mean values, open circles are data from individual experiments;n=12). (d) Effect of Ihblock onEGABA(A)(filled circles are mean values, open circles are data from individual experiments;n=12). (e) Summary graph showing the effect of ZD-7288 onEGABA(A)andVR.EGABA(A)became more depolarized thanVRin 10 out of 12 cells (open circles: control, filled circles: in ZD-7288). Error bars represent s.e.m.; *P<0.05, **P<0.01. Figure 4: Blocking I h changes the V R – E GABA(A) relationship in CA1 pyramidal cells. ( a ) In control conditions, all cells had negative E GABA(A) compared with V R ( n =12). Sample IPSPs at different membrane potentials from a typical experiment are shown in the inset. Data points were fitted with a second-order polynomial function. ( b ) Time course of the changes in V R following the application of ZD-7288 ( n =12). ( c ) Effect of ZD-7288 on V R (filled circles are mean values, open circles are data from individual experiments; n =12). ( d ) Effect of I h block on E GABA(A) (filled circles are mean values, open circles are data from individual experiments; n =12). ( e ) Summary graph showing the effect of ZD-7288 on E GABA(A) and V R . E GABA(A) became more depolarized than V R in 10 out of 12 cells (open circles: control, filled circles: in ZD-7288). Error bars represent s.e.m. ; * P <0.05, ** P <0.01. Full size image Correcting V R after I h block restores coincidence detection Although the broadening of input integration is consistent with the hypothesis that GABA A receptor-mediated hyperpolarization is required to maintain the narrow time window for coincidence detection, an alternative potential explanation is that I h has a profound effect upon dendritic excitability and temporal summation of excitatory inputs [12] , [13] . To distinguish between these hypotheses, we repeated the coincidence-detection experiments, but depolarized the neuron following addition of ZD-7288 to return the resting membrane potential to the baseline level. Using this protocol, we observed no change in the time window for integration ( Fig. 5 ; n =5; repeated measures ANOVA: F (1,4)=0.374, P =0.57). This implies that it is primarily the depolarizing effect of I h and loss of the hyperpolarizing effect of GABA A receptor currents that maintains the narrow coincidence detection for input integration. A further prediction from this is that simple hyperpolarization with I h intact would widen the coincidence-detection time window, which is indeed the case ( n =5, repeated measures ANOVA: F(1,4)=8.2, P =0.046; Supplementary Fig. S3 ). 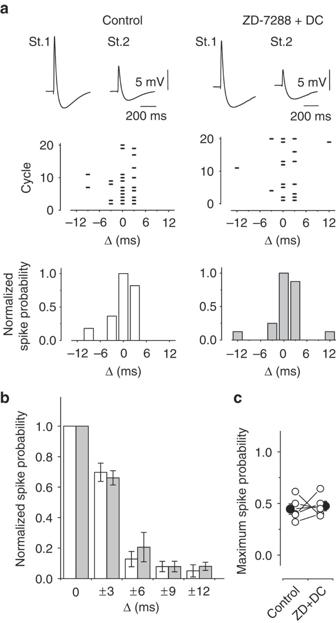Figure 5: Repolarization restores temporal precision when Ihis blocked. (a) Spike probability at different intervals between stimuli in control conditions and in the presence of ZD-7288 when neurons were repolarized to their initialVRby DC injection, therefore restoring the biphasic shape of the EPSP–IPSP sequence. Top: sample traces; middle: raster plots of spikes initiated by stimulation of the two pathways at different delay intervals; bottom: spike probability distribution graphs. (b) Averaged data from five experiments (open columns: control, shaded columns: ZD-7288+DC;P=0.57). (c) Probability of action potential generation for synchronous stimulation of both pathways before and after application of ZD-7288 (n=5). Error bars represent s.e.m. Figure 5: Repolarization restores temporal precision when I h is blocked. ( a ) Spike probability at different intervals between stimuli in control conditions and in the presence of ZD-7288 when neurons were repolarized to their initial V R by DC injection, therefore restoring the biphasic shape of the EPSP–IPSP sequence. Top: sample traces; middle: raster plots of spikes initiated by stimulation of the two pathways at different delay intervals; bottom: spike probability distribution graphs. ( b ) Averaged data from five experiments (open columns: control, shaded columns: ZD-7288+DC; P =0.57). ( c ) Probability of action potential generation for synchronous stimulation of both pathways before and after application of ZD-7288 ( n =5). Error bars represent s.e.m. Full size image Hyperpolarizing inhibition underlies temporal precision A possible confounder in the above experiments is that in order to maintain a 50% spiking probability, we had to adjust the stimulation intensity to compensate for the membrane hyperpolarization, potentially affecting interneuron recruitment. This would tend to increase the interneuron recruitment and therefore would be expected to narrow the integration time window (in contrast to the broadening that we observed). Nevertheless, to control for this and to address the question of whether loss of the hyperpolarization effect of GABA A receptor currents is sufficient to explain our results, we constructed a simple integrate-and-fire model of a neuron that receives two inputs. Each input consisted of an excitatory followed by an inhibitory conductance, and the parameters were adjusted to simulate the kinetics of the experimentally obtained EPSP–IPSP sequence waveform (see Methods ; Fig. 6a ). In agreement with the experimental findings, systematic variation of the delay between the two inputs revealed a narrow integration time window for spike generation ( Fig. 6b ). 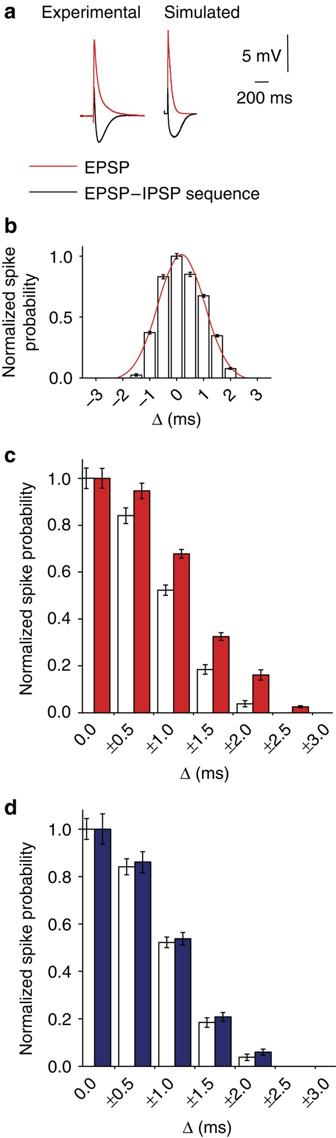Figure 6: Ih-mediated hyperpolarization broadens the integration time window in an integrate-and-fire neuronal model. (a) Successive activation of excitatory and inhibitory conductances in a simple integrate-and-fire neuron was used to produce an EPSP–IPSP sequence similar to that observed experimentally. (b) Simulation of two pathways activated with different delays (seeMethods) resulted in a narrow integration time window. Synaptic strength was adjusted so that the peak probability of action potential generation remained at 50%. (c) Removal of Ihfrom the dendrites hyperpolarized the modelled neuron by 10 mV. The graph shows spike probability at different intervals between stimuli with (open bars) and without Ih(red bars) in the modelled neuron. (d) The effect of Ihremoval was abolished when the neuronal soma was repolarized by DC injection (open bars: control with Ih, blue bars: no Ihrepolarized). Data are presented as means of 30 rounds of simulations, error bars represent s.e.m. Figure 6: I h -mediated hyperpolarization broadens the integration time window in an integrate-and-fire neuronal model. ( a ) Successive activation of excitatory and inhibitory conductances in a simple integrate-and-fire neuron was used to produce an EPSP–IPSP sequence similar to that observed experimentally. ( b ) Simulation of two pathways activated with different delays (see Methods ) resulted in a narrow integration time window. Synaptic strength was adjusted so that the peak probability of action potential generation remained at 50%. ( c ) Removal of I h from the dendrites hyperpolarized the modelled neuron by 10 mV. The graph shows spike probability at different intervals between stimuli with (open bars) and without I h (red bars) in the modelled neuron. ( d ) The effect of I h removal was abolished when the neuronal soma was repolarized by DC injection (open bars: control with I h , blue bars: no I h repolarized). Data are presented as means of 30 rounds of simulations, error bars represent s.e.m. Full size image Hyperpolarization of V R broadens the integration time window Removing I h from the modelled cell, hyperpolarized the membrane from −70 to −80 mV and led to an increase in the width of the integration time window ( Fig. 6c ; the area under the spike probability curve was increased by 26.3±2.3%; P <0.01). This effect was robust and relatively insensitive to varying EPSP and IPSP kinetic parameters, delay times between excitatory and inhibitory synapse activation, as well as synapse locations on the dendrites ( Supplementary Fig. S4 ). We also systematically changed the maximal probability of action potential generation to test whether this could affect our experimental results. The effect of membrane potential hyperpolarization was constant across a wide range of tested probability values ( Supplementary Fig. S5 ). To determine whether the effect on the integration window in the simulations was due to the conductance or voltage effect of I h removal, we repolarized the neuronal soma back to −70 mV by introducing a depolarizing current. In agreement with experimental observations, this restored the width of the time window for integration, indicating a crucial role for the depolarizing action of I h ( Fig. 6d ). We next asked whether the effect that we observed was due to the voltage change itself rather than the change in the polarity of GABA A receptor-mediated transmission. We therefore assessed the effects of membrane potential on the integration time window in the absence of GABAergic transmission. As expected [4] , removing feed-forward inhibition broadened the integration time window by 106.8±6.7%. However, the width of the window was minimally affected by changes in V R in the range observed in our experiments and simulations ( Fig. 7a ; an increase of 3.1±0.4% with 10 mV hyperpolarization). 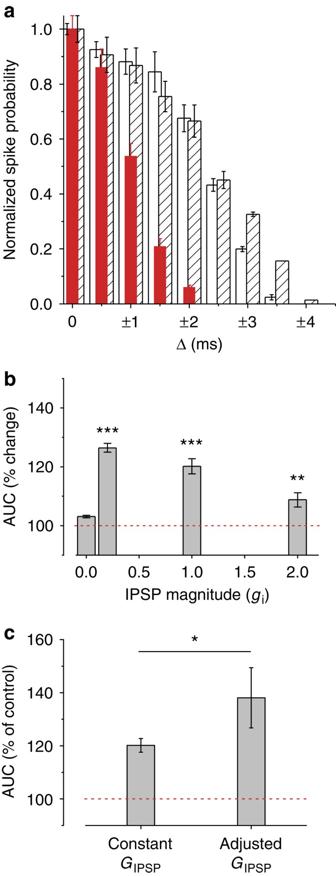Figure 7: The effects of changing the magnitude of inhibitory conductances on the width of the integration time window. (a) In the absence of feed-forward inhibition (no IPSPs), the integration time window became broader. Under such conditions, membrane hyperpolarization did not change the width of coincidence detection, indicating that changes in the polarizing effect of GABAAreceptor-mediated currents, rather than theVRvalue itself, determine neuronal integration (open bars:Vm=−70 mV no IPSP; hatched bars:Vm=−80 mV no IPSP; red bars:Vm=−70 mV with IPSP). (b) The effect of varying the strength of inhibitory connections on the width of the integration time window assessed as the change in the area under the spike probability curve (AUC). (c) The effect of hyperpolarization on the coincidence-detection time window when inhibitory synaptic conductances were scaled with excitatory conductances, mimicking the situation when inhibitory inputs onto a neuron are not saturated. Data are presented as means of 30 rounds of simulations, error bars represent s.e.m.; *P<0.05, **P<0.01, ***P<0.001. Figure 7: The effects of changing the magnitude of inhibitory conductances on the width of the integration time window. ( a ) In the absence of feed-forward inhibition (no IPSPs), the integration time window became broader. Under such conditions, membrane hyperpolarization did not change the width of coincidence detection, indicating that changes in the polarizing effect of GABA A receptor-mediated currents, rather than the V R value itself, determine neuronal integration (open bars: V m =−70 mV no IPSP; hatched bars: V m =−80 mV no IPSP; red bars: V m =−70 mV with IPSP). ( b ) The effect of varying the strength of inhibitory connections on the width of the integration time window assessed as the change in the area under the spike probability curve (AUC). ( c ) The effect of hyperpolarization on the coincidence-detection time window when inhibitory synaptic conductances were scaled with excitatory conductances, mimicking the situation when inhibitory inputs onto a neuron are not saturated. Data are presented as means of 30 rounds of simulations, error bars represent s.e.m. ; * P <0.05, ** P <0.01, *** P <0.001. Full size image In the above simulations, the magnitude of the inhibitory synaptic conductance was fixed to match the simulated EPSP–IPSP waveform with that observed experimentally. We therefore tested the effect of different inhibitory synaptic conductances. In all instances, hyperpolarizing V R , so that the IPSPs became depolarizing, widened the integration time window. This effect initially increased with increases in the IPSP amplitude ( Fig. 7b ) up to a maximum and then decreased probably because of the increasing shunting versus voltage effect of inhibitory synapses. Finally, we considered the possible confounding effect of variability in the size of the inhibitory conductance. At high stimulation intensity, the inhibitory conductance is relatively invariant [29] . However, at lower stimulation intensities, inhibitory conductances vary with stimulation intensity (and magnitude of excitatory conductance). We therefore covaried the conductances of excitatory and inhibitory synapses (see Methods ) to model this situation. Under these conditions, the window of integration was still increased following hyperpolarization of the neuron by 38.1±11.4% compared with 20.2±2.6%, with constant inhibitory synaptic conductances ( Fig. 7c ; P <0.05). We have shown that I h is necessary to maintain a hyperpolarizing driving force for GABA A receptor-mediated transmission by depolarizing the resting membrane potential of pyramidal cells. Hyperpolarizing the resting membrane potential through pharmacological inhibition of I h or deletion of HCN1 results in depolarizing GABA A receptor-mediated potentials and broadening of the excitatory phase of the EPSP–IPSP sequence, leading to a prolonged time window for synaptic integration. These results also demonstrate an important and unexpected role of voltage inhibition. I h channels are densely expressed in the dendritic arbour of CA1 pyramidal cells [21] . A significant proportion of these channels is active at rest, reducing the membrane resistance and neuronal time constant. These effects of I h have been shown to determine the time course of EPSPs onto CA1 pyramidal cells [12] . The previous studies have concentrated on the impact of I h on the integration properties of excitatory inputs, with GABA A receptor-mediated inhibition blocked. However, GABAergic inhibition has a profound effect on the width of the integration time window of excitatory inputs [4] . The relative roles of shunting and hyperpolarizing inhibition in maintaining precise coincidence detection have not been addressed. Although one study has considered the effect of I h on the integration time window without GABA A receptor blockade [6] , that work was performed in whole-cell mode, with the membrane potential of the neurons fixed and the reversal potential of GABA A responses set to be depolarizing. In hippocampal neurons, E GABA(A) is negative to V R by the end of the second postnatal week [30] , so that GABA A receptor-mediated potentials predominantly hyperpolarize the postsynaptic membrane in adult tissue, for example, see ref. ( 31 ). In adult neurons, E GABA(A) is mainly determined by the Cl − cotransporter KCC2, which uses the transmembrane K + gradient to maintain a low intracellular Cl − concentration, thereby clamping the reversal potential for Cl − ( E Cl ) closer to that of K + ( E K ) [30] . E GABA(A) is, however, more depolarized than E Cl due to the permeability of the GABA A receptors to HCO 3 − ions [32] . Therefore, to maintain hyperpolarizing IPSPs, V R also has to be depolarized relative to E GABA(A) . A number of conductances may contribute to this depolarization (such as persistent sodium currents and leak conductances); in CA1 pyramidal cells, I h provides a significant depolarizing drive at resting membrane potential [11] . In our study, this effect of I h was more evident with pharmacological block than with genetic ablation, perhaps because of compensatory changes in other conductances in the HCN1 knockout mice. We have shown that I h sets the polarity of GABAergic events by making V R more depolarized than E GABA(A) , and most of the effects of I h on the EPSP–IPSP sequence can be rescued by repolarizing V R to its baseline value, arguing for a major role of GABAergic voltage inhibition in regulating the integration properties of synaptic inputs of CA1 pyramidal cells. As observed in our study and in other studies, for example, see ref. ( 33 ), GABA A receptor activation can still shunt EPSPs even when E GABA(A) is more depolarized than V R . However, the relative importance of shunting and hyperpolarizing effects of inhibition for neuronal computations and precise timing of action potential generation has received much less attention. Some experimental and theoretical studies have suggested that the hyperpolarizing effects of GABAergic neurotransmission are critical for network synchronization, for example, see ref. ( 34 ), whereas others emphasize the role of shunting inhibition in oscillatory behaviour of interconnected neurons [35] . The ability of I h to switch the inhibitory mode of GABAergic signals from hyperpolarizing to shunting or depolarizing adds further complexity in defining the computational properties of hippocampal neurons [36] . Further, it might be expected that the large, early shunting effect of GABAergic inhibition has the predominant part in curtailing the EPSPs. Our results, however, underscore the contribution of GABA A receptor-mediated hyperpolarization in determining the temporal precision of coincidence detection by hippocampal pyramidal neurons. How does changing the GABA A receptor-mediated response from hyperpolarizing translate to an increased integration time? Although shunting is maintained regardless of the polarization of GABA A receptor-mediated responses (see Fig. 2a ) attenuating the EPSPs generated in response to the second stimulation, this attenuation would be much stronger when the IPSP produces hyperpolarization. More importantly, because the voltage effect of an IPSP outlasts its shunting effect [33] , it would have an impact on the excitatory potentials over an extended period. In the situation when the hyperpolarizing phase of the GABAergic response is abolished (and even more so if the polarity of the GABA A response is changed), this would facilitate EPSP summation. Therefore, the hyperpolarization that results from inhibition of I h results in a considerable increase in the half-width of the time window for coincidence detection. Inhibition of other membrane conductances through hyperpolarization cannot account for this, as voltage changes of similar magnitudes, when I h is blocked, result in minimal change in the membrane resistance or time constant [11] . The critical role of hyperpolarization for coincidence detection has extensive implications, as anything that alters the polarity of GABA A receptor-mediated transmission will affect the time window for input integration. This would include either a shift in E GABA(A) (for example, due to loss or inhibition of KCC2) or changes in resting membrane potential mediated through, for example, changes in membrane potassium conductances. We have therefore shown the critical role of GABA A receptor-mediated hyperpolarization in information processing and an unexpected mechanism by which I h can modulate coincidence detection. As I h is regulated by developmental [37] , physiological [38] and pathological processes [16] , [39] , [40] , [41] , [42] , such processes may consequently affect the properties of GABA A receptor-mediated signalling and the temporal fidelity of coincidence detection. This may contribute to cognitive and psychiatric consequences of epilepsy by increasing the probability of aberrant associations. Moreover, the magnitude of somatic I h is dependent upon excitatory synaptic activity, and this has been proposed to be a homeostatic mechanism regulating neuronal excitability [38] . We further hypothesize that such a mechanism may have an additional homeostatic role by narrowing the time window for coincidence detection with increases in neuronal activity and conversely broadening the time window for integration when synaptic activity decreases. The role of I h in restricting temporal input integration may also contribute to explaining the enhanced learning behaviour observed in HCN1 knockout mice [27] , which may occur at the expense of loss of temporal discrimination of inputs. Electrophysiology We used transverse hippocampal slices (350 μm) from 3–6-week-old male Sprague–Dawley rats, or HCN1 knockout mice and their wild-type littermate controls. The HCN1 knockout animals were re-derived from that described previously, and maintained on a 129SVEV background [27] , [28] . Animals were killed according to schedule 1 of the UK Animals (Scientific Procedures) Act 1986. The brains were rapidly removed, dissected and cut with Leica VT1000S vibratome in ice-cold solution containing (in mM) sucrose (70), NaCl (80), KCl (2.5), MgCl 2 (7), CaCl 2 (0.5), NaHCO 3 (25), NaH 2 PO 4 (1.25) and glucose (22), and were equilibrated with 95% O 2 /5% CO 2 (pH 7.4). The slices were allowed to recover in an interface chamber (>1 h) at room temperature before being transferred to the recording chamber. Storage and perfusion solutions contained (in mM) NaCl (119), KCl (2.5), MgSO 4 (1.3), CaCl 2 (2.5), NaHCO 3 (26.2), NaH 2 PO 4 (1) and glucose (22), and were gassed with 95% O 2 /5% CO 2 . All recordings, except for those in Figures 1 , 5 and Supplementary Figure S3 , were carried out at 32 °C. Current-clamp whole-cell recordings ( Supplementary Fig. S1 ) were performed using pipettes (3–5 MΩ) filled with an intracellular solution containing (in mM) K-gluconate (145), NaCl (8), KOH–HEPES (10), EGTA (0.2), Mg-ATP (2) and Na 3 -GTP (0.3); pH 7.2; 290 mOsm. Gramicidin (50 μg ml −1 ) was added for perforated-patch recordings [43] , and patch pipettes (8–12 MΩ) were front-filled with gramicidin-free solution; either QX-314 Br (5 mM) was added or [Cl − ] was increased to 26 mM ( E Cl =−41 mV) to monitor patch integrity. Series resistance was monitored throughout. Data acquisition began when the series resistance was <150 MΩ (15–20 min after obtaining cell-attached configuration). To isolate GABA A receptor-mediated IPSPs, NMDA, AMPA and GABA B receptors were blocked with AP5 (50 μM), NBQX (20 μM) and CGP52432 (5 μM), respectively. Constant current stimuli were delivered to Schaffer collaterals through bipolar stainless steel electrodes placed in stratum radiatum. Monosynaptic IPSPs were evoked by positioning the stimulating electrode close to the recording site. EPSP–IPSP sequences were evoked by positioning the electrodes in stratum radiatum at least 300 μm away from the recording site; CGP52432 (5 μM) was added to the perfusate. Although application of CGP52432 reduced the duration of the hyperpolarizing phase by 16±3% ( Supplementary Fig. S6a–c ), it did not affect the depolarizing component. Two Schaffer collateral pathways were stimulated for the coincidence-detection protocol ( Figs 1 and 5 , Supplementary Fig. S3 ). Experiments were performed in the presence of 50 μM AP5 (to avoid spike timing-dependent plasticity) and 5 μM CGP52432. AP5 had a minimal impact on the excitatory phase of the EPSP–IPSP sequence, decreasing the half-width by 14±4% (more than an order of magnitude smaller than the impact of changing the polarity of GABA A responses; Supplementary Fig. S6d–f ). To ensure recording stability, these experiments were performed at room temperature (23–25 °C); this increased the time course of the synaptic responses ( Supplementary Fig. S7 ), but the shape of the EPSP–IPSP waveform was maintained. Although modelling indicated that this does not qualitatively change the experimental findings ( Supplementary Fig. S4a ), we confirmed this with cell-attached recordings at 32 °C ( Supplementary Fig. S2 ). These experiments were performed using patch pipettes (8–12 MΩ) filled with ACSF in voltage-clamp with the voltage set so that no current was injected under baseline conditions. As afferent input strength to the hippocampus can vary considerably, we stimulated a weak and a strong input; the amplitude of the response in one pathway was adjusted to be approximately twice than that in the other pathway. In the cell-attached experiments, the 'weak' pathway was stimulated at approximately half-threshold intensity, whereas the 'strong' pathway stimulation was set close to the firing threshold. Stimulation intensities were adjusted to obtain ∼ 50% spike probability when the two pathways were activated simultaneously. The two pathways were stimulated with an interstimulus delay varying from −12 to +12 ms in 3 ms steps (thus the order of inputs was reversed over the range investigated). To avoid any confounding effects of asymmetric distribution of spike probabilities, the data are presented as the averaged values from corresponding points on either side of the maximum. In some experiments, constant current injection was used to repolarize the somatic membrane potential. Under our experimental conditions, there is a space clamp error in distal dendrites. However, as we observed experimentally that somatic current injection restored the hyperpolarization phase of the EPSP–IPSP waveform, we conclude that feed-forward inhibition in our study was predominantly perisomatic ( Supplementary Fig. S8 ). For experiments on the effect of I h block on the magnitude of IPSCs, the intracellular solution contained (in mM) Cs-methanesulfonate (120), NaCl (8), HEPES (10), EGTA (0.2), MgCl 2 (0.2), Mg-ATP (2), Na 3 -GTP (0.3) and QX-314 Br (5 mM); 290 mOsm. Schaffer collaterals were stimulated in the presence of AP5 and CGP52432. Neurons were voltage-clamped at 0 mV (close to the reversal potential for AMPA receptor-mediated response), and outward GABA A receptor-mediated currents were compared in the absence and presence of ZD-7288. All recordings were obtained using a MultiClamp 700B amplifier (Molecular Devices), filtered at 2 kHz and digitized at 5 kHz. LabView (National Instruments) software was used for data acquisition and off-line analysis. Chemicals were purchased from Tocris Cookson or Sigma-Aldrich. Modelling All simulations were conducted with NEURON 7.0 (ref. 44 ) on a multimode cluster 45 . The Hodgkin–Huxley neuron model consisted of a cylindrical soma (diameter=length=20 μm) and two identical dendrites (3 μm diameter and 200 μm long). The axial resistance ( R a ) was 35.4 Ohm cm −1 ; membrane capacitance ( C m ) was 1 μF cm −2 . The somatic membrane had Na + and K + conductances with the following peak values: g Na =0.12 S cm −2 , g K =0.036 S cm −2 ( E K =−77 mV and E Na =+50 mV). The dendritic membrane had a passive leak current ( g pas =1 mS cm −2 and E pas =−80 mV) and I h ( g Ih =1 mS cm −2 , kinetics as in ref. 21 ). V R was −70 mV. Removal of I h hyperpolarized the neuron by 10 mV. In such conditions, 0.4 nA injected into the soma was necessary to repolarize the membrane potential to −70 mV. All simulations were performed with either V R =−70 mV (baseline conditions) or −80 mV (hyperpolarized conditions). Deterministic action potential generation was prevented by introducing Poisson-distributed conductances of uniformly distributed variable magnitude (0.9–1.1 nS; τ rise =0.1 ms; τ decay =1 ms; reversal potential= V R to avoid significant membrane potential fluctuations) into the cell at a mean frequency of 1,000 Hz. Each dendrite had a glutamatergic and GABAergic synapses, located at 180 and 40 μm from the soma, respectively. The dual-exponential formalism in the Exp2Syn function of neuron simulator was used to determine the time course of synaptic conductances: where g s ( t ) is the synaptic conductance at time t after activation; τ 1 is the rise time constant (7 ms for glutamatergic synapses and 15 ms for GABAergic synapses); τ 2 is the decay time constant (35 ms for glutamatergic synapses and 50 ms for GABAergic synapses) and G m is the value of the maximum synaptic conductance. To simulate the EPSP–IPSP sequence, there was a 7 ms delay from EPSPs to IPSPs. The reversal potentials were set at −75 and 0 mV for GABAergic and glutamatergic synapses, respectively. The left excitatory and inhibitory synaptic conductances ( G ESL and G ISL ) were twice the right synaptic conductances ( G ESR and G ISR ). The onset time of the left EPSP–IPSP sequence was fixed whereas that of the right varied from −10 to +10 ms. To calculate the time distribution of the spike probability, interstimulus intervals were divided into 0.5 ms bins. The probability of action potential generation was determined using 30 rounds of ten synaptic stimulations with 500 ms interval between trials, initiated with a different seed. The interval between stimuli was sufficient to allow the model neuron to reach initial steady-state conditions. The mean number of action potentials per bin ( M i ) and s.e. ( ɛ i ) were calculated. Area under the spike probability curve was used to quantify changes in the coincidence-detection time window. The s.e. of the surface under the distribution was defined as: where N is the number of bins, bin is the bin size and p max is the maximum probability of the distribution. The s.e. of the ratio of surfaces S1/S2 was defined as: The maximal probability of action potential generation (0.5) was set by scaling synaptic conductances with the parameter Stim: Stim× G ESL and Stim× G ESR . The strengths of inhibitory synapses were set to G ISL =450 nS and G ISR =225 nS for left and right synapse, respectively, for the majority of simulations. For Figure 7b , the strength of inhibitory connections varied as indicated. For simulations presented in Figure 7c in addition to excitatory conductances, we also scaled inhibitory conductances: Stim× G ISL and Stim× G ISR . Simulations with maximal probabilities from 0.2 to 0.85 were performed ( Supplementary Fig. S5 ). In these experiments, the actual maximal spike probability was determined post hoc . Statistics Two-tailed Student's t -test (paired or independent) and repeated measures ANOVA were used for statistical analysis. P <0.05 for significant differences. Data are presented as mean±s.e.m. How to cite this article: Pavlov, I. et al . I h -mediated depolarization enhances the temporal precision of neuronal integration. Nat. Commun. 2:200 doi: 10.1038/ncomms1202 (2011).